Endohedral fullerene with μ3-carbido ligand and titanium-carbon double bond stabilized inside a carbon cage In all metallofullerenes known before this work, metal atoms form single highly polar bonds with non-metal atoms in endohedral cluster. This is rather surprising for titanium taking into account the diversity of organotitanium compounds. Here we show that the arc-discharge synthesis of mixed titanium-lutetium metallofullerenes in the presence of ammonia, melamine or methane unexpectedly results in the formation of TiLu 2 C@ I h -C 80 with an icosahedral I h (7) carbon cage. Single-crystal X-ray diffraction and spectroscopic studies of the compound reveal an unprecedented endohedral cluster with a μ 3 -carbido ligand and Ti-C double bond. The Ti(IV) in TiLu 2 C@ I h -C 80 can be reversibly reduced to the Ti(III) state. The Ti=C bonding and Ti-localized lowest unoccupied molecular orbital in TiLu 2 C@ I h -C 80 bear a certain resemblance to titanium alkylidenes. TiLu 2 C@ I h -C 80 is the first metallofullerene with a multiple bond between a metal and the central, non-metal atom of the endohedral cluster. One of the unique properties of fullerenes is their ability to encapsulate metal atoms with the formation of endohedral metallofullerenes (EMFs) [1] , [2] , [3] , [4] . In EMFs, the metals donate their valence electrons to the carbon cage and adopt large positive charges. Therefore, when two or more metal atoms are encapsulated in one fullerene molecule, they experience strong Coulomb repulsion. This destabilizing interaction can be balanced by the formation of clusterfullerenes [5] , which are EMFs whose endohedral clusters also include non-metals (for example, N, (ref. 6 ) O, (ref. 7 ) S, (ref. 8 ) C 2 (ref. 9 )). So far, most clusterfullerenes are based on the trivalent metals such as Sc, Y and lanthanides. Thus, the formal charge distribution in the molecules of the most abundant class of EMFs, nitride clusterfullerenes (NCFs) M 3 N@C 2 n , can be described as (M 3+ ) 3 N 3− @C 2 n 6− (ref. 10 ). The frontier molecular orbitals (MOs) in NCFs are usually localized on the carbon cage, and hence the metal atoms in NCFs are inert and their trivalent state is not amenable to variation by chemical or electrochemical means [11] , [12] . The notable exceptions are Ti-based NCFs, TiSc 2 N@ I h -C 80 and TiY 2 N@ I h -C 80 (refs 13 , 14 , 15 ). The nitride cluster works as a template to enforce a trivalent state of an endohedral Ti atom, which can be then oxidized or reduced to the Ti IV and Ti II states [13] . In addition to the Ti-NCFs, the only known Ti-EMFs are Ti@C 28 (seen only in the gas phase so far) [16] , the carbides Ti 2 C 2 @C 78 and Ti 2 C 2 @C 82 (refs 17 , 18 ), and a sulphide Ti 2 S@C 78 (ref. 19 ). In all Ti-EMFs known before this work, Ti formed single highly polar bonds with non-metal atoms in the clusters. For example, the intracluster bonding in Ti 2 C 2 @C 78 can be described as Ti–C≡C–Ti. Thus, the bonding mode of Ti in EMFs is not different from Sc, Y and lanthanides, which is rather surprising taking into account a diversity of organotitanium compounds [20] , [21] . In addition to titanocenes, Ti is able to form single, double and triple Ti˙˙˙C bonds. Since the invention of the Ziegler–Natta process of olefin polymerization, many Ti-based organometallic complexes have been used as catalysts of industrial importance. For instance, compounds with Ti=C double bonds of the general formula L 2 Ti=CR 2 (where L is a ligand and R is H or alkyl) known as Schrock carbenes or alkylidenes are widely used in olefination reactions [22] , [23] , [24] , [25] , [26] . Ti in L 2 Ti=CR 2 is usually a 16-electron system with LUMO localized on the metal. Due to such an electronic structure, L 2 Ti=CR 2 molecules are very unstable in the pristine form and readily coordinate other groups to Ti or decompose [27] . As a result, (Cp) 2 Ti=CR 2 species are frequently formed only in situ as transient intermediates [28] , [29] . For example, the archetypical Schrock carbene (Cp) 2 Ti=CH 2 is usually obtained from the Tebbe reagent (Cp) 2 TiCH 2 (Cl)Al(CH 3 ) 2 (ref. 30 ), Grubbs’ titanocyclobutane [31] , or Petasis reagent (Cp) 2 Ti(CH 3 ) 2 (ref. 32 ). So far, (Cp) 2 Ti=CH 2 was detected only by mass-spectrometry [33] , whereas X 2 Ti=CH 2 (X=H, F, Cl) species were isolated in low-temperature inert gas matrices [34] , [35] . At the same time, Ti alkylidenes with a higher coordination number, when Ti-based LUMO is further coordinated, can form stable molecules [22] , [23] , [36] , [37] , [38] , [39] . In this work we report on a new type of Ti-EMFs which have a double Ti=C bond and μ 3 -carbido ligand in the TiLu 2 C cluster. Although Ti here is a 16-electron system with Ti-localized LUMO similar to the (Cp) 2 Ti=CR 2 species, the structure is stabilized by encapsulation of the TiLu 2 C cluster in the C 80 carbon cage. Synthesis of TiLu 2 C 81 The title compound was first obtained in the arc-discharge synthesis with the use of Lu 2 O 3 /Ti 2 O 3 and NH 3 as a reactive gas. Under these conditions, the formation of empty fullerenes and conventional EMFs is suppressed yielding Lu 3 N@C 2 n NCFs as the main fullerene products (see Fig. 1a ). The mixed-metal Ti-Lu EMF was obtained as a minor product, however, its mass-spectrum was different from the expected nitride clusterfullerene TiLu 2 N@C 80 and the composition was identified as TiLu 2 C 81 . Similar results were obtained when melamine (C 3 N 6 H 6 ) was used as the solid source of nitrogen instead of gaseous NH 3 ( Fig. 1b ). Melamine also partially suppresses formation of empty fullerenes and leads to NCFs as the main products. In contrast to the NH 3 -assisted synthesis, melamine also resulted in the formation of appreciable amounts of Lu 2 @C 82 and Lu 2 C 2 @C 82 . TiLu 2 N@C 80 was not formed at all, and TiLu 2 C 81 was the main Ti-containing EMF produced. In both the NH 3 - and the melamine-directed syntheses, TiLu 2 C 81 is the main component of the fraction isolated at a retention time of 35.6–37.5 min. On the basis of chromatographic peak areas, the relative yield of TiLu 2 C 81 versus Lu 3 N@ I h -C 80 in the synthesis with NH 3 and melamine is estimated as 1 and 3%, respectively. 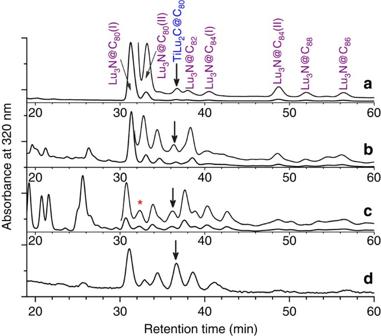Figure 1: Chromatograms of the raw Ti-Lu fullerene extracts. (a) synthesis with NH3, (b) synthesis with melamine, (c) synthesis with molecular nitrogen, (d) synthesis with methane as a reactive gas. The arrow indicates the fraction containing TiLu2C81, the red asterisk marks the fraction containing TiLu2N@C80. Figure 1: Chromatograms of the raw Ti-Lu fullerene extracts. ( a ) synthesis with NH 3 , ( b ) synthesis with melamine, ( c ) synthesis with molecular nitrogen, ( d ) synthesis with methane as a reactive gas. The arrow indicates the fraction containing TiLu 2 C 81 , the red asterisk marks the fraction containing TiLu 2 N@C 80 . Full size image In the view of the unexpected formation of TiLu 2 C 81 and the absence of TiLu 2 N@C 80 in the conditions favourable for the synthesis of NCFs, arc synthesis was performed in the presence of molecular nitrogen under conditions used by Yang et al. to synthesize TiSc 2 N@C 80 and TiY 2 N@C 80 (refs 14 , 15 ). This procedure indeed resulted in the formation of TiLu 2 N@C 80 , but TiLu 2 C 81 was also found among the products ( Fig. 1c ). Since TiLu 2 C 81 does not contain nitrogen, the synthesis was also performed in the absence of any nitrogen source with a He atmosphere. However, no TiLu 2 C 81 was detected in such conditions. The best method for the synthesis of TiLu 2 C 81 was found to be a reactive atmosphere method with methane such as the method used in our group earlier to synthesize Sc 3 CH@C 80 (ref. 40 ). Arc-discharge synthesis in the presence of CH 4 yields TiLu 2 C 81 as one of the main EMF products ( Fig. 1d ) along with Lu 3 N@ I h -C 80 (formed presumably because of the traces of nitrogen in methane and generator) and some Lu 2 @C 2 n and Lu 2 C 2 @C 2 n compounds. Isolation of pure TiLu 2 C 81 in the methane-based synthesis can be accomplished in one high-performance liquid chromatography (HPLC) step, since TiLu 2 C 81 is the main component of the fraction eluted at 36–38 min. Molecular structure of TiLu 2 C@ I h -C 80 The isolation of pure TiLu 2 C 81 (see Fig. 2a for its mass-spectrum) enabled the elucidation of its molecular structure. Two lines in a 3:1 intensity ratio in the 13 C NMR spectrum of TiLu 2 C 81 at 136.82 and 143.67 p.p.m. ( Fig. 2b ) unambiguously show that this endohedral metallofullerene utilizes the icosahedral I h (7)-C 80 carbon cage with a freely rotating endohedral cluster (for comparison, the 13 C lines of Lu 2 ScN@ I h -C 80 are found at 137.12 and 143.99 p.p.m. [41] ). Thus, the formula of TiLu 2 C 81 can be written as TiLu 2 C@ I h -C 80 . Unfortunately, even after accumulation of the spectrum over two weeks, the signal of the central carbon atom could not be observed. 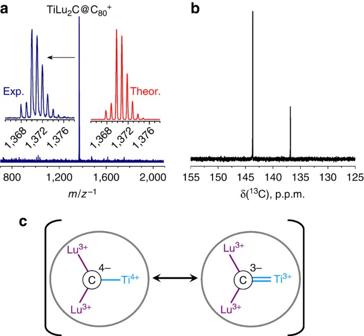Figure 2: Spectroscopic identification of TiLu2C@Ih-C80. (a) LDI mass-spectrum of TiLu2C@Ih-C80with experimental and calculated isotopic distribution; (b)13C NMR spectrum of TiLu2C@Ih-C80; (c) schematic description of the electronic distribution in TiLu2C@Ih-C80. exp., experimental; LDI, laser desorption ionization; theor., theoretical. Figure 2: Spectroscopic identification of TiLu 2 C@ I h -C 80 . ( a ) LDI mass-spectrum of TiLu 2 C@ I h -C 80 with experimental and calculated isotopic distribution; ( b ) 13 C NMR spectrum of TiLu 2 C@ I h -C 80 ; ( c ) schematic description of the electronic distribution in TiLu 2 C@ I h -C 80 . exp., experimental; LDI, laser desorption ionization; theor., theoretical. Full size image The molecular structure of TiLu 2 C@ I h -C 80 was obtained by single-crystal X-ray diffraction as shown in Fig. 3 . The asymmetric unit of TiLu 2 C@ I h -C 80 ·Ni(OEP)·2(toluene) has no crystallographically imposed symmetry and consists of independent molecules of each of the four components. A typical host–guest interaction occurs between the fullerene and the porphyrin. Also, the two toluenes exhibit face-to-face interaction with the fullerene. The shortest contact between the central Ni atom of the host porphyrin and the cage is Ni1 … C1, 2.871(5) Å. The existence of a central, single carbide (C81) was indicated by the increase in agreement factors when C is replaced by N ( R 1 increases from 0.0578 to 0.0580). Further indications stem from the overall geometric features. Four orientations for TiLu 2 were refined. Their relative orientations are shown in Supplementary Fig. 1a . The major orientation of the TiLu 2 unit has a fractional occupancy of 0.6475(15). Occupancies of three other minor sites are 0.1747(12), 0.1126(12) and 0.0651(12). Positional disorder in the central carbon position (C81) was not detected but it is likely to exist in correlation with the minor three groups. 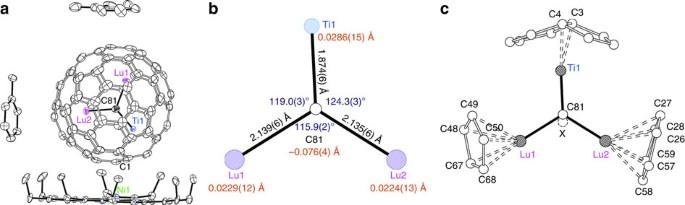Figure 3: Single-crystal X-ray structure of TiLu2C@Ih-C80. (a) A view of the structure of TiLu2C@Ih-C80·Ni(OEP)·2(toluene) with hydrogen atoms omitted for clarity; only the predominant Ti and Lu positions are shown. Displacement parameters are shown at the 50% probability level. (b) The structure of the major TiLu2C cluster with X-ray determined bond lengths and bond angles. The numbers in red are the displacements of the atoms from the plane of the TiLu2C unit. (c) The view showing the interactions of the metal ions with the closest portions of the cage. The dotted circle marked X represents the centre of the C80cage. Figure 3: Single-crystal X-ray structure of TiLu 2 C@ I h -C 80 . ( a ) A view of the structure of TiLu 2 C@ I h -C 80 ·Ni(OEP)·2(toluene) with hydrogen atoms omitted for clarity; only the predominant Ti and Lu positions are shown. Displacement parameters are shown at the 50% probability level. ( b ) The structure of the major TiLu 2 C cluster with X-ray determined bond lengths and bond angles. The numbers in red are the displacements of the atoms from the plane of the TiLu 2 C unit. ( c ) The view showing the interactions of the metal ions with the closest portions of the cage. The dotted circle marked X represents the centre of the C 80 cage. Full size image Although there is disorder in the position of the TiLu 2 unit, it is fortunate that there is a dominant site with large population. Due to uncertainty in the minor positions, only the major site (65%) for the TiLu 2 C interior group should be taken as representative of the cluster geometry, and our discussion of the structure will focus on this dominant site. In it, the Ti1–C81 distance is short, at 1.874(6) Å. The Lu–C distances of 2.135(6) and 2.139(6) Å are longer than the Lu–N distances previously found for Lu 3 N@ I h -C 80 (range, 2.00–2.07 Å) [42] . In TiLu 2 C@ I h -C 80 , the trimetallic unit is nearly planar; C81 is 0.076(4) Å from the least-squares plane of the TiLu 2 C unit. The sum of the angles about C81 is 359.2°. The dihedral angle between the porphyrin plane and the TiLu 2 C plane is 82.3°. Also, the edge of the TiLu 2 C plane is not between the two N-Ni-N lines but rather lies approximately parallel to one of them ( Supplementary Fig. 1b ). This arrangement is in agreement with what is observed in the M 3 N@ I h -C 80 metal porphyrin structures [43] . As seen in (c) in Fig. 3 , each metal atom has a different interaction with the carbon cage, and those of Ti are particularly short. Notably, C81 is displaced by 0.33 Å from the cage centroid in the direction of Ti1, and Ti1 has the shortest cage contacts. Ti1 is centred on a 5:6 ring junction with Ti1˙˙˙C3 and Ti1˙˙˙C4 distances of 2.137(6) and 2.150(6) Å, respectively. Lu1 is η 5 to a pentagon with Lu˙˙˙C distances in the range from 2.309(6) to 2.678(6) Å; Lu2 is η 6 to a hexagon with Lu˙˙˙C distances in the range 2.318(5) to 2.563(6) Å. Further evidence for the strong cage interaction with Ti can be seen in the very large pyramidalization angles [44] of 13.7° at C3 and C4. Only C67 has a larger pyramidalization angle, 13.8°, corresponding to the shortest Lu1˙˙˙C distance. For comparison, the remaining 77 carbon pyramidalization angles average 9.9° (see Supplementary Fig. 2 ). The charge distribution in TiLu 2 C might be written as a carbide [(Lu 3+ ) 2 Ti 4+ C 4− ] 6+ , as shown in Fig. 2c . Note that Ti 4+ C 4− fragment is isoelectronic to Sc 3+ N 3− , and hence TiLu 2 C@ I h -C 80 has certain analogy to nitride clusterfullerene Lu 2 ScN@ I h -C 80 . However, structural and computational studies and the vibrational spectroscopy discussed below show that a more appropriate description of the cluster structure is [(Lu 3+ ) 2 Ti 3+ =C 3− ] 6+ with a double bond between the titanium and the central carbon atom ( Fig. 2c ). The length of the Ti=C bond in TiLu 2 C@ I h -C 80 , 1.874(6) Å, falls into the range of the Ti=C bond lengths in Ti alkylidenes characterized by single-crystal X-ray diffraction (usually 1.8–1.9 Å, see Supplementary Table 1 for a list of values) [22] , [23] . The structure of the planar TiLu 2 C cluster with μ 3 -carbido ligand bonded to three metal atoms is rather unusual and has only few analogues in organometallic chemistry, and none of them involves Ti [45] , [46] , [47] , [48] . For instance, Floriani et al. reported the structure in which μ 3 -C is bonded to two Nb and one Na ions [45] , whereas Matsuzaka et al. synthesized a Ru 2 Pt complex with μ 3 -carbido ligand [46] . The carbon-metal bonds in these clusters have double bond character and resemble the bonding in corresponding alkylidenes. DFT calculations of the molecular structure and bonding Deeper insight into the molecular and electronic structure of TiLu 2 C@ I h -C 80 was obtained by DFT computations and topological analysis of the electronic density using Quantum Theory of Atoms in Molecules (QTAIM) [49] . In agreement with the fast rotation of the cluster that was revealed by 13 C NMR spectroscopy, computations showed the existence of several orientational conformers of the TiLu 2 C cluster inside the I h -C 80 cage in the energy range of 0–10 kJ mol −1 (see Supplementary Fig. 3 and Supplementary Table 2 ). A similar situation is also found for group III nitride clusterfullerenes (for example, Lu 2 ScN@ I h -C 80 ) [10] , [11] , [12] , [41] in contrast to TiM 2 N@ I h -C 80 (M=Sc, Y, Lu), which show more enhanced dependence of the relative energy on the cluster position [13] , [14] , [15] . The DFT predicted Ti=C bond length in TiLu 2 C@ I h -C 80 is 1.836 Å, ~0.04 Å shorter than experimental value. For comparison, the length of the single Ti–C bond in Ti 2 C 2 @C 78 predicted at the same level of theory is 1.976 Å (see Table 1 for some other relevant bond lengths). Table 1 Selected QTAIM parameters for L 2 Ti=CH 2 , TiLu 2 C@ I h -C 80 , and other EMFs*. Full size table To learn more about the bonding situation in the TiLu 2 C cluster as well as the metal–cage bonding, we applied a topological QTAIM analysis. In this work we focus mainly on the QTAIM atomic charges and delocalization indices δ(A,B) which denote the number of electron pairs shared between the atoms A and B. For non-polar bonds, δ(A,B) values have the physical meaning of bond orders in Lewis definition, whereas for polar bonds, the values are reduced compared with the formal bond order. The sum of all δ(M, C) indices for a given metal atom M and carbon atoms from the carbon cage defines a ‘metal-cage bond order’ [50] . Table 1 compares selected QTAIM parameters for clusterfullerenes TiLu 2 C@ I h -C 80 , TiLu 2 N@ I h -C 80 , Lu 2 ScN@ I h -C 80 , Ti 2 C 2 @C 78 , as well as methylidenes L 2 Ti=CH 2 (L=Cp, Cl, and F). An analysis of the bond critical point indicators (electron density, Laplacian, energy densities and so on) is given in Supplementary Table 3 . Depending on the ligand L, the DFT-optimized Ti=C bond lengths in these L 2 Ti=CH 2 species vary from 1.849 Å (Cl) to 1.951 Å (Cp), whereas the δ(Ti, C) values are changing inversely with the bond length from 1.34 (Cp) to 1.71 (Cl). Note that the δ(Ti, C) values are smaller than 2 in all L 2 Ti=CH 2 molecules because of the significant polarity of the Ti=C bond (according to atomic charges, Ti donates 0.60–0.66 e to the carbon atom of the =CH 2 group). QTAIM parameters of the Ti=C bond in TiLu 2 C@ I h -C 80 , including the δ(Ti, C) index, atomic charge of Ti, as well as the number of electron pairs shared with the π-ligands, are strikingly similar to those of Cp 2 Ti=CH 2 . Besides, the δ(Ti, C) value in TiLu 2 C@ I h -C 80 is approximately two times higher than δ(Sc/Lu, N) values in nitride clusterfullerenes as well as the δ(Ti, C) index for a single Ti–C bond in Ti 2 C 2 @C 78 . These data show that the description of the carbon-titanium bond by a C 4− –Ti 4+ charge distribution is not appropriate and should be done in terms of double polar C 3− =Ti 3+ bond. At the same time, the large negative charge of the central carbon atom in TiLu 2 C@ I h -C 80 is very similar to that of the nitrogen atom in NCFs, showing their nucleophilic nature. Thus, QTAIM analysis supports the formal charge distribution depicted in Fig. 2 and clearly shows that the Ti=C bond in TiLu 2 C@ I h -C 80 can be described as a double bond similar to that in Ti alkylidenes (see Supplementary Note 1 and Supplementary Table 3 for further comparison of the Ti–C bond in the TiLu 2 C cluster and in Ti alkylidenes). Vibrational spectra Detailed information on the intracluster as well as metal–cage interactions can be obtained by means of vibrational spectroscopy. In line with the close similarity of their molecular structures, the Fourier transform infrared spectra of Lu 2 ScN@ I h -C 80 (ref. 51 ) and TiLu 2 C@ I h -C 80 ( Fig. 4 ) exhibit a pronounced similarity in the ranges dominated by the carbon cage vibrations (400–600, 1,000–1,600 cm −1 ). 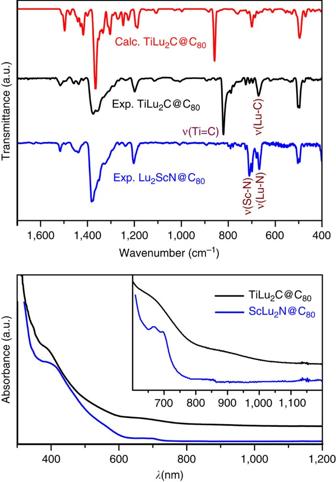Figure 4: FTIR and UV–vis-NIR spectra of TiLu2C@Ih-C80and LuSc2N@Ih-C80. Top: room-temperature FTIR spectra on KBr substrate and DFT-computed IR spectrum of TiLu2C@Ih-C80. Bottom: UV–vis-NIR absorption spectra of TiLu2C@Ih-C80and Lu2ScN@Ih-C80in toluene solution. calc., calculated; DFT, density dunctional theory; exp., experimental; FTIR, Fourier transform infrared (spectroscopy); NIR, near infrared; UV, ultraviolet. Figure 4: FTIR and UV–vis-NIR spectra of TiLu 2 C@ I h -C 80 and LuSc 2 N@ I h -C 80 . Top: room-temperature FTIR spectra on KBr substrate and DFT-computed IR spectrum of TiLu 2 C@ I h -C 80 . Bottom: UV–vis-NIR absorption spectra of TiLu 2 C@ I h -C 80 and Lu 2 ScN@ I h -C 80 in toluene solution. calc., calculated; DFT, density dunctional theory; exp., experimental; FTIR, Fourier transform infrared (spectroscopy); NIR, near infrared; UV, ultraviolet. Full size image The main difference between the spectra of two EMFs in the mid-IR range is found for the metal-nitrogen anti-symmetric stretching modes of Lu 2 ScN@ I h -C 80 (denoted as ν(M–N) hereafter) and analogous vibrations of TiLu 2 C@ I h -C 80 . In M 3 N@C 80 species, the ν(M–N) mode is two-fold degenerate and corresponds to the motions of the nitrogen atom in the plane of the M 3 N cluster [52] . In the mixed-metal nitride cluster such as Lu 2 ScN, the ν(M–N) mode is split: the higher-frequency component (near 710 cm −1 ) corresponds to the vibration with the dominant contribution of the Sc–N stretching, whereas the lower-frequency component (at 667 cm −1 ) has mainly a ν(Lu–N) character [51] . The lower mass of the carbon atom should result in the 8% upshift of the vibrational frequencies of the ν(M–C) modes in the TiLu 2 C cluster if the M–C and M–N force constants are equal. However, Lu–C bonds in the TiLu 2 C@ I h -C 80 are noticeably longer than the Lu–N bonds in Lu 2 ScN@ I h -C 80 (2.178 Å versus 2.147 Å in DFT-optimized structure). As the increase of the bond length results in the downshift of its vibrational frequency, the force constant and mass factors in TiLu 2 C@ I h -C 80 compensate, and the ν(Lu–C) mode is found at 670 cm −1 , very close to the frequency of the ν(Lu–N) mode in Lu 2 ScN@ I h -C 80 . On the contrary, the ν(Ti=C) mode in TiLu 2 C@ I h -C 80 is found at 821 cm −1 , which is 16% higher than the frequency of the ν(Sc–N) mode in Lu 2 ScN@ I h -C 80 . Obviously, this large shift is caused both by the lower mass of the carbon atom and by a much shorter Ti=C bond in comparison to the Sc−N bond in Lu 2 ScN@ I h -C 80 (1.836 Å versus 1.945 Å). Note also that the ν(Ti=C) frequency in TiLu 2 C@ I h -C 80 is considerably higher than the ν(Ti=C) frequencies of the matrix-isolated F 2 Ti=CH 2 and Cl 2 Ti=CH 2 species found at 706 and 680 cm −1 , respectively [34] , [35] , which is consistent with the short bond length given by crystal results. Similar to the IR spectra, the regions of the Raman spectra of two EMFs corresponding to the cage vibrations exhibit a pronounced similarity ( Supplementary Fig. 4 ). For the analysis of the cluster–cage interactions, the most informative one is the low-frequency range of 100–200 cm −1 comprising vibrations of the endohedral clusters ( Supplementary Fig. 4 ).The modes corresponding to the metal–cage interaction are found at approximately the same frequencies both in Lu 2 ScN@C 80 and TiLu 2 C@C 80 showing that cluster–cage interactions are similar in these EMFs in agreement with the same extent of the cluster-to-cage electron transfer (see Supplementary Note 2 for more detailed analysis of the Raman spectra). Electronic structure of TiLu 2 C@ I h -C 80 Figure 4 compares the absorption spectra of TiLu 2 C@ I h -C 80 and Lu 2 ScN@ I h -C 80 measured in toluene solution. Absorption spectra of EMFs correspond to the π→π* excitations of the carbon cage and hence the spectra of all M 2 ScN@ I h -C 80 species are very similar and closely resemble those of M 3 N@ I h -C 80 (M=Y and lanthanides) [51] . The absorption onset of Lu 2 ScN@C 80 is observed near 800 nm, and the lowest energy absorption features are distinguished at 666 and 691 nm followed by more intense bands at 558 and 402 nm ( Fig. 4 , also see ref. 51 ). In the visible range, the spectrum of TiLu 2 C@ I h -C 80 with the main features at 390 nm and near 540 nm also resembles that of Lu 2 ScN@ I h -C 80 , however, the bands are broader and less defined. At the 600–700 nm range, TiLu 2 C@ I h -C 80 exhibits only one broad absorption band at 670 nm (versus two better resolved features in Lu 2 ScN@ I h -C 80 ). The main difference between the two EMFs is found in the lowest energy range: whereas Lu 2 ScN@ I h -C 80 has no well-defined absorptions beyond 700 nm, TiLu 2 C@ I h -C 80 exhibits one weak band at 910 nm, and its absorption onset is extended to ~1,100 nm. On the basis of the onset and lowest energy absorption, the lowest and highest estimations of the bandgap of TiLu 2 C@ I h -C 80 can be determined as 1.13 and 1.36 eV, respectively, which is ~0.4 eV smaller than analogous values determined for Lu 2 ScN@ I h -C 80 (1.55–1.79 eV). Thus, absorption spectra reveal that in spite of the same electron count and similar nature of the cluster–cage interactions, the electronic properties of TiLu 2 C@ I h -C 80 are noticeably different from those of Lu 2 ScN@ I h -C 80 . On the basis of the frontier MO analysis (see below), the lowest energy excitation in TiLu 2 C@ I h -C 80 can be presumably assigned to the cage-to-Ti electron transfer. 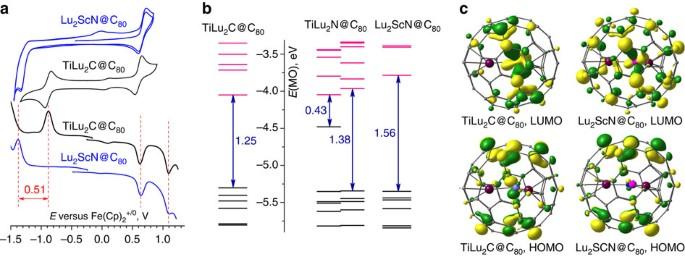Figure 5: Frontier MO analysis of TiLu2C@Ih-C80and Lu2ScN@Ih-C80. (a) Cyclic voltammetry and square wave voltammetry (SWV) curves of TiLu2C@Ih-C80(black lines) and Lu2ScN@Ih-C80(blue lines); (b) Kohn–Sham MO energy levels (occupied—black, unoccupied—pink) of TiLu2C@Ih-C80, TiLu2N@Ih-C80and Lu2ScN@Ih-C80; (c) isosurfaces of the frontier MOs of TiLu2C@Ih-C80and Lu2ScN@Ih-C80. Figure 5a compares the results of the cyclic voltammetry and square wave voltammetry studies of TiLu 2 C@ I h -C 80 and Lu 2 ScN@ I h -C 80 , and Table 2 lists the measured redox potentials. At room temperature in o -dichlorobenzene ( o -DCB) solution, TiLu 2 C@ I h -C 80 exhibits one reversible reduction and one reversible oxidation step at −0.91 and +0.63 V, respectively, (versus the Fc(Cp) 2 +/0 couple) resulting in an electrochemical gap of 1.54 V. Figure 5: Frontier MO analysis of TiLu 2 C@ I h -C 80 and Lu 2 ScN@ I h -C 80 . ( a ) Cyclic voltammetry and square wave voltammetry (SWV) curves of TiLu 2 C@ I h -C 80 (black lines) and Lu 2 ScN@ I h -C 80 (blue lines); ( b ) Kohn–Sham MO energy levels (occupied—black, unoccupied—pink) of TiLu 2 C@ I h -C 80 , TiLu 2 N@ I h -C 80 and Lu 2 ScN@ I h -C 80 ; ( c ) isosurfaces of the frontier MOs of TiLu 2 C@ I h -C 80 and Lu 2 ScN@ I h -C 80 . Full size image Table 2 Redox potentials of TiLu 2 C@ I h -C 80 , Lu 2 ScN@ I h -C 80 and selected relevant EMFs*. Full size table The reversible reduction of TiLu 2 C@ I h -C 80 is quite remarkable, since NCFs with group III metals (including Lu 2 ScN@ I h -C 80 ) exhibit electrochemically irreversible reductions [2] , [53] . The electrochemical behaviour of TiLu 2 C@ I h -C 80 at the first reduction step is similar to that of other Ti-based EMFs, such as diamagnetic Ti 2 S@C 78 , paramagnetic TiSc 2 N@C 80 and TiY 2 N@C 80 , which exhibit reversible reductions at −0.92, −0.94 and −1.11 V, respectively, and all EMFs are characterized by the reduction localized at the Ti atom [13] , [15] , [19] . Note also that the Ti(III)/Ti(IV) oxidation potential of Ti-alkylidene (Nacnac)Ti(CH 2 t Bu) 2 in THF reported by Mindiola et al. is −0.90 V (Nacnac − =[Ar]NC(Me)CHC(Me)N[Ar], Ar=2,6-(CHMe 2 ) 2 C 6 H 3 ) (ref. 37 ). The cyclic voltammogram of Lu 2 ScN@ I h -C 80 measured under the same conditions as TiLu 2 C@ I h -C 80 exhibits an irreversible reduction at −1.41 V (peak potential), which is 0.50 V more negative than the first reduction potential of TiLu 2 C@ I h -C 80 . On the contrary, the first oxidation of Lu 2 ScN@ I h -C 80 is reversible and occurs at +0.66 V, very close to the oxidation potential of TiLu 2 C@ I h -C 80 (+0.63 V). Interestingly, oxidation potentials of TiM 2 N@ I h -C 80 are found at much more negative values (+0.16 and 0.00 V for M=Sc and Y, respectively). Note also that redox potentials of Lu 2 ScN@ I h -C 80 are close to those of Lu 3 N@ I h -C 80 (ref. 54 ). Frontier MO analysis Experimental studies reveal that the bandgap of TiLu 2 C@ I h -C 80 is 0.4–0.5 eV smaller than that of the isoelectronic Lu 2 ScN@ I h -C 80 because the former has a lower-energy LUMO presumably localized on Ti. On the contrary, HOMO of TiLu 2 C@ I h -C 80 has a similar energy to that of Lu 2 ScN@ I h -C 80 . These conclusions are further rationalized by the DFT-based frontier orbital analysis. Figure 5 shows MO energy levels in TiLu 2 C@ I h -C 80 , TiLu 2 N@ I h -C 80 and Lu 2 ScN@ I h -C 80 as well as the isosurfaces of the HOMOs and LUMOs. The LUMO of TiLu 2 C@ I h -C 80 is largely localized on the Ti atom resembling that of Cp 2 Ti=CH 2 and is 0.27 eV below the LUMO energy of Lu 2 ScN@ I h -C 80 . The latter also has a similar shape to the LUMO of TiLu 2 C@ I h -C 80 , but the carbon cage contribution to the MO is much larger at the expense of the lower Sc contribution. The shapes and the energies of the HOMOs of TiLu 2 C@ I h -C 80 and Lu 2 ScN@ I h -C 80 are almost identical, and both MOs are essentially carbon cage orbitals. MO analysis also explains a similar reductive and different oxidative behaviour of TiLu 2 C@ I h -C 80 and Ti-NCFs. Figure 5 shows that the lowest energy vacant MO of the TiLu 2 N@C 80 at −3.96 eV has almost the same energy as the LUMO of TiLu 2 C@ I h -C 80 (−4.05 eV) and hence their reduction potentials should be similar. On the contrary, oxidation of TiLu 2 N@ I h -C 80 (as well as other TiM 2 N@ I h -C 80 ) removes one electron from the Ti-based SOMO, whose energy is well above the HOMO energy of TiLu 2 C@ I h -C 80 . Hence, oxidation potentials of Ti-NCFs are much lower than that of TiLu 2 C@ I h -C 80 . Further details of MO analysis focusing on the intracluster bonding are given in Supplementary Fig. 5 and Supplementary Note 3 . In this work we have discovered a new type of endohedral clusterfullerenes with central μ 3 -C atom and double Ti=C bond. The Ti-C bonding in TiLu 2 C@ I h -C 80 and metal-based LUMO resembles those in the unstable L 2 Ti=CR 2 carbenes with 16-electron Ti (such as Cp 2 Ti=CH 2 ). However, unlike the latter, TiLu 2 C@ I h -C 80 is stable at the room temperature (in toluene solution kept in the dark, the sample did not show any traces of decomposition over the period of 1.5 years), which can be ascribed to the protective role of the fullerene cage. Finally, TiLu 2 C@ I h -C 80 was fully characterized by spectroscopic and electrochemical techniques and its electronic structure was found to be intermediate between that of conventional M III -based nitride clusterfullerenes M 3 N@ I h -C 80 and nitride clusterfullerenes with one Ti atom, TiM 2 N@ I h -C 80 . Synthesis of TiLu 2 C@C 80 with the use of NH 3 Mixed-metal cluster fullerenes were produced by evaporating graphite rods in the electric arc in the Krätschmer–Huffman method modified in our group. The graphite rods (length 100 mm, diameter 8 mm) were packed with Lu 2 O 3 , Ti 2 O 3 , and graphite (molar ratio of Lu:Ti:C=1:1:15) and evaporated in 200 mbar helium atmosphere with addition of ammonia (20 mbar NH 3 ) with the current of 100 A. The soot produced by arc vaporization was first pre-extracted with acetone for one hour to remove non-fullerene products and then Soxhlet extracted for 20 h with carbon disulphide. At the first step, isolation of the fractions containing Lu 3 N@C 2n and TiLu 2 C@C 80 was accomplished by HPLC using analytical 4.6 mm × 250 mm Buckyprep column (Nacalai Tesque, Japan) and toluene as a solvent. The fraction collected at 35.64–37.49 min was then subjected to the second purification step by recycling HPLC at the BuckyPrep column (toluene as eluent, flow rate 1.5 ml min −1 ). See Supplementary Fig. 6 for HPLC traces and mass-spectrum. Synthesis of TiLu 2 C@C 80 with the use of other reagents The synthesis with molecular nitrogen was performed using the same procedure as described for NH 3 above, except for the use of an inert He atmosphere (200 mbar) with addition of N 2 (20 mbar) instead of NH 3 (see Supplementary Fig. 7 for HPLC trace and mass-spectra). The synthesis with melamine was performed using similar procedure, except for the use of an inert He atmosphere (200 mbar) and pure metals (not their oxides). The ratio of the components in the packed rods was Lu:Ti:C:N=1:1:15:10. HPLC traces and mass-spectrum are shown in Supplementary Fig. 8 . In the synthesis with methane, the total pressure was 250 mbar (238 mbar He and 12 mbar CH 4 ), the ratio of components in the packed rods was Lu:Ti:C=1:1:12.5. Spectroscopic measurements Laser desorption time-of-flight mass-spectra were measured using Biflex III (Bruker, Germany). The 125 MHz 13 C NMR spectra were measured at room temperature in carbon disulphide solutions with d 6 -acetone as a lock on an Avance 500 spectrometer (Bruker, Germany) using the multiprobe head PH 1152Z. Ultraviolet–vis-near-infrared absorption spectra were measured at room temperature in toluene solution on a Shimadzu 3100 spectrophotometer. The Fourier transform infrared spectra were recorded at room temperature in transmission mode by a Vertex 80v spectrometer (Bruker, Germany) with a resolution of 2 cm −1 . Raman spectra were recorded at 78 K on a T 64000 triple spectrometer (Jobin Yvon, France) with visible laser radiation (Innova 300 series, Coherent, USA). For IR and Raman measurements, the sample was drop-coated onto single-crystal KBr disks. The residual toluene was removed by heating the polycrystalline films in vacuum at 200 °C for 3 h. Single-crystal X-ray diffraction Black blocks were obtained by slow diffusion of a toluene solution of the endohedral fullerene into a toluene solution of Ni(OEP). A crystal suitable for X-ray diffraction was mounted in the nitrogen cold stream at 100(2) K provided by an Oxford Cryostream low-temperature apparatus on the goniometer head of a Bruker D8 diffractometer equipped with an ApexII CCD detector at the Advanced Light Source, Berkeley, California, beamline 11.3.1. Data were collected with the use of silicon(111) monochromated synchrotron radiation ( λ =0.77490 Å). The data set was reduced with the use of Bruker SAINT (Bruker AXS Inc., Madison, Wisconsin, USA) and a multi-scan absorption correction applied with the use of SADABS [55] . The structures were solved by direct methods (SHELXS-2013 (ref. 55 )) and refined by full-matrix least-squares on F 2 (SHELXL-2013 (ref. 55 )). Crystal data: C 131 H 60 Lu 2 N 4 NiTi, fw=2146.38, triclinic, space group P -1, a =14.6351(7) Å, b =14.6452(7) Å, c =20.4465(10), α =83.295(3), β =83.193(3), γ =60.662(3), V =3784.7(3) Å 3 , Z =2, 75,518 data, R (int)=0.0568; R 1 (24,183 reflections with I >2σ( I ))=0.0578, wR 2 (all 28,472 data=0.1563, 1,343 parameters, 19 restraints. Further details of crystal refinement are described in Supplementary Note 4 . Electrochemistry Voltammetric experiments were performed with a PAR 273 potentiostat (EG&G, USA) at room temperature in a glove box. A three-electrode system using a platinum working and a counter electrode and a silver wire reference electrode was used. Potentials were measured by adding ferrocene as an internal standard. Computations Optimization of the structures was performed at the PBE [56] level using Priroda [57] , [58] package and implemented basis set of TZ2P quality with effective core potential for Ti and Lu atoms. For QTAIM and MO analyses, point energy computations were performed at the PBE level with full-electron TZVP basis set and ZORA correction implemented in ORCA code [59] , [60] . QTAIM analysis was performed using AIMAll suite ( http://aim.tkgristmill.com/ ). Accession codes The X-ray crystallographic coordinates for structures reported in this article have been deposited at the Cambridge Crystallographic Data Centre (CCDC), under deposition number CCDC 980876. These data can be obtained free of charge from The Cambridge Crystallographic Data Centre via www.ccdc.cam.ac.uk/data_request/cif . How to cite this article: Svitova, A. L. et al. Endohedral fullerene with μ 3 -carbido ligand and Titanium-Carbon double bond stabilized inside a carbon cage. Nat. Commun. 5:3568 doi: 10.1038/ncomms4568 (2014).